Adaptive synonymous mutations in an experimentally evolvedPseudomonas fluorescenspopulation Conventional wisdom holds that synonymous mutations, nucleotide changes that do not alter the encoded amino acid, have no detectable effect on phenotype or fitness. However, a growing body of evidence from both comparative and experimental studies suggests otherwise. Synonymous mutations have been shown to impact gene expression, protein folding and fitness, however, direct evidence that they can be positively selected, and so contribute to adaptation, is lacking. Here we report the recovery of two beneficial synonymous single base pair changes that arose spontaneously and independently in an experimentally evolved population of Pseudomonas fluorescens. We show experimentally that these mutations increase fitness by an amount comparable to non-synonymous mutations and that the fitness increases stem from increased gene expression. These results provide unequivocal evidence that synonymous mutations can drive adaptive evolution and suggest that this class of mutation may be underappreciated as a cause of adaptation and evolutionary dynamics. Synonymous mutations might be expected to have no detectable effect on fitness, as this class of mutation does not change the amino-acid sequence of the encoded protein. However, it has been recognized for sometime that this assumption may not always be correct. Pervasive variation in the frequencies of synonymous codons across genes and genomes (codon usage bias) [1] suggests that selection may favour some synonymous codons over others. Moreover, direct measures of the impact of synonymous mutations from nucleotide replacement studies demonstrate that they can impact gene expression [2] , [3] , presumably through changes to the rate or accuracy of transcription and/or translation [4] , mRNA stability and folding [5] , protein secondary structure [6] , [7] and even fitness [3] , [8] , [9] , [10] , [11] . Taken together, these results suggest that the frequency of at least some synonymous mutations is governed by selection. The nature of selection on synonymous mutations—its direction and strength—is less clear. Theory suggests that the strength of selection on synonymous sites resulting in observed patterns of codon bias is probably weak, on the order of 1/ N e ( N e : effective population size) for genes with intermediate levels of codon bias and up to ~2/ N e for genes with extreme codon bias [12] . Consistent with this expectation, estimates of fitness from comparative genomics suggest that synonymous sites are under weak purifying selection [13] , [14] , [15] , although a recent study suggests that up to 22% of synonymous sites in the Drosophila melanogaster genome may be under strong purifying selection [16] . Direct measures of fitness from site-directed mutagenesis studies tell a similar story: the fitness effects of synonymous mutations are almost always deleterious or, more rarely, weakly beneficial [3] , [8] , [9] , [10] , [11] . Deleterious mutations are, by definition, subject to purifying selection, while weakly beneficial mutations are unlikely to be substituted by selection because either they cannot escape drift in small populations or, in large populations, are eliminated in competition with the relatively more abundant class of non-synonymous mutations with larger beneficial effects. The occasional recovery of synonymous mutations from microbial evolution experiments could imply that they are under positive selection, but often little focus is given to these mutations (for example, see ref. 17 ), the assumption being that they have hitch hiked to high frequency alongside a genetically linked beneficial non-synonymous substitution. Further investigation of the fitness effects associated with synonymous mutations from these experiments typically reveals that these mutations are indeed neutral [18] , [19] . Taken together, the evidence suggests that the fitness effects of synonymous mutations are most often either nearly neutral or deleterious and, very infrequently, weakly beneficial. Such variability in fitness effects suggests that we might be able to describe the distribution of fitness effects among synonymous mutations in much the same way as we do for any other kind of mutation, including non-synonymous ones: the distribution should be modal, with a mean that is on average negative and a right-hand tail that encompasses at least some beneficial mutations. If this interpretation is correct, then we should occasionally expect to see strongly beneficial synonymous mutations that are positively selected and contribute to adaptation. To date, however, direct evidence that such mutations exist is lacking. Here we report the recovery of two independently arising beneficial synonymous mutations driving adaptive evolution in a laboratory population of the Gram-negative bacterium, Pseudomonas fluorescens . These mutations have strong beneficial fitness effects, comparable to the fitness effects of beneficial non-synonymous mutations arising in similar experimental populations, that are caused by increased gene expression at the level of transcription and can be common in natural populations. Our results suggest that synonymous mutations may play an underappreciated role in adaptive evolution. Substitution dynamics of synonymous mutations As part of a larger experiment [20] , we propagated an initially isogenic population of P. fluorescens strain SBW25 for 1,000 generations in a minimal medium containing glucose as the sole carbon source. Fitness was assayed every 200 generations and increased significantly by 14.79% ( t -test, df=2, P =0.01939) relative to the ancestor by the end of the experiment ( Fig. 1a ). Comparing whole-genome sequences of the generation 1000 population with the ancestor revealed two synonymous single base pair changes in the putatively annotated gtsB (PFLU4845) gene (A15A: GCA→GCG; G38G: GGC→GGT; see Fig. 2a ) and a 35,107 bp deletion, Δ(PFLU4435–4466). We reconstructed the dynamics of substitution by isolating 24 colonies every 200 generations and probing each isolate for the relevant mutation ( Fig. 1a,b ). The Δ(PFLU4435–4466) genotype appeared first around generation 200 and was nearly fixed by generation 400 before being replaced by a second genotype with the gtsB (A15A) mutation in the Δ(PFLU4435–4466) background, which rose to high frequency by generation 800 and was itself nearly replaced by the Δ(PFLU4435–4466) gtsB (G38G) genotype by the end of the experiment. This pattern, with each new genotype arising and nearly fixing within 200 generations, is consistent with natural selection acting on strongly beneficial mutations. 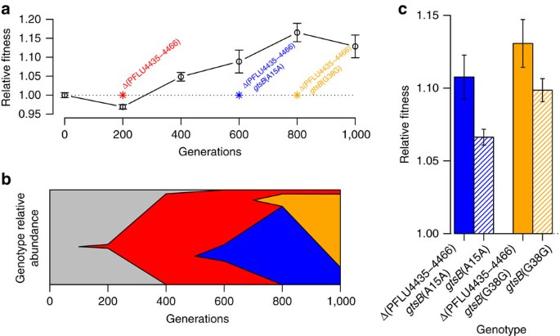Figure 1: Fitness and genotype trajectories of aP. fluorescenspopulation adapting to glucose minimal media over 1,000 generations. (a) Population fitness relative to the ancestor (SBW25), over 1,000 generations (mean±s.e.m.;n=3); * indicates when genotypes were first detected. (b) Relative abundance of the ancestor (grey), Δ(PFLU4435–4466) (red), Δ(PFLU4435–4466)gtsB(A15A) (blue), Δ(PFLU4435–4466)gtsB(G38G) (yellow) genotypes over 1,000 generations. (c) Fitness of the evolved genotypes (solid bars) and the synonymous mutations in the ancestral genetic background (hashed bars) relative to the ancestor (mean±s.e.m.;n=8). Figure 1: Fitness and genotype trajectories of a P. fluorescens population adapting to glucose minimal media over 1,000 generations. ( a ) Population fitness relative to the ancestor (SBW25), over 1,000 generations (mean±s.e.m. ; n =3); * indicates when genotypes were first detected. ( b ) Relative abundance of the ancestor (grey), Δ(PFLU4435–4466) (red), Δ(PFLU4435–4466) gtsB (A15A) (blue), Δ(PFLU4435–4466) gtsB (G38G) (yellow) genotypes over 1,000 generations. ( c ) Fitness of the evolved genotypes (solid bars) and the synonymous mutations in the ancestral genetic background (hashed bars) relative to the ancestor (mean±s.e.m. ; n =8). 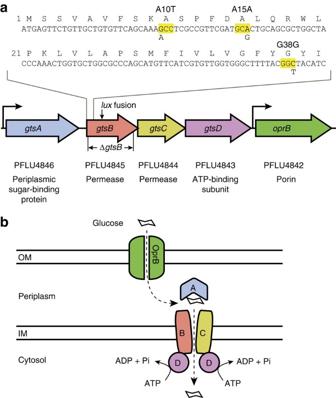Figure 2: Genomic and functional context of the synonymous (A15A and G38G) and non-synonymous (A10T) substitutions. (a) The substitutions occurred in the 5′ region of PFLU4845, which encodes a permease subunit of an ATP-binding cassette (ABC) transporter. The DNA and amino-acid sequence of the first 40 codons are shown, with the nucleotide substitutions indicated below the highlighted codons. Neighbouring genes encode three additional ABC transporter subunits and an outer membrane porin. The transporter gene names (gts, glucose transporter subunit) are based on those of theP. putidaKT2440 homologues23. The open reading frame lengths, position of the luciferase (lux) transcriptional fusion junction and ΔgtsB-deleted region are drawn to scale. Bent arrows indicate promoters predicted by the Softberry BPROM program (http://linux1.softberry.com/berry.phtml). (b) The schematic depicts the probable subunit organization of the gene products during glucose uptake40. Glucose crosses the outer membrane by facilitated diffusion through the OprB porin, interacts with the periplasmic glucose-binding protein (GtsA) and is transported across the inner membrane channel (GtsBCD2) in a process energized by ATP hydrolysis. IM, inner membrane; OM, outer membrane. Full size image Figure 2: Genomic and functional context of the synonymous (A15A and G38G) and non-synonymous (A10T) substitutions. ( a ) The substitutions occurred in the 5′ region of PFLU4845, which encodes a permease subunit of an ATP-binding cassette (ABC) transporter. The DNA and amino-acid sequence of the first 40 codons are shown, with the nucleotide substitutions indicated below the highlighted codons. Neighbouring genes encode three additional ABC transporter subunits and an outer membrane porin. The transporter gene names ( gts , glucose transporter subunit) are based on those of the P. putida KT2440 homologues [23] . The open reading frame lengths, position of the luciferase ( lux ) transcriptional fusion junction and Δ gtsB- deleted region are drawn to scale. Bent arrows indicate promoters predicted by the Softberry BPROM program ( http://linux1.softberry.com/berry.phtml ). ( b ) The schematic depicts the probable subunit organization of the gene products during glucose uptake [40] . Glucose crosses the outer membrane by facilitated diffusion through the OprB porin, interacts with the periplasmic glucose-binding protein (GtsA) and is transported across the inner membrane channel (GtsBCD 2 ) in a process energized by ATP hydrolysis. IM, inner membrane; OM, outer membrane. Full size image Beneficial fitness effects of synonymous mutations Assays of competitive fitness confirm that both evolved genotypes containing the synonymous substitutions confer a significant fitness advantage over the ancestor and, moreover, that Δ(PFLU4435–4466) gtsB (G38G) is fitter than Δ(PFLU4435–4466) gtsB (A15A) ( Fig. 1c ), consistent with the substitution dynamics observed ( Fig. 1a,b ). To estimate the fitness effect of the synonymous mutations themselves, we used an allelic replacement strategy to introduce each synonymous mutation into the ancestral genetic background that lacked the Δ(PFLU4435–4466) mutation (see Methods). Competitive fitness assays reveal that gtsB (A15A) confers a 7.25% (±0.55 s.e.m.) and gtsB (G38G) a 8.73% (±0.79 s.e.m.) fitness advantage relative to the ancestor ( Fig. 1c ), values that are substantially larger than any previous estimate of fitness for a synonymous mutation [3] , [8] , [9] , [10] , [11] . Confirmation that gtsB is a target of selection The intensity and breadth of resource use that these mutations confer provides insight into the ultimate causes of selection. Four lines of evidence suggest that these mutations were selected because of their fitness advantage on glucose rather than general adaptation to laboratory conditions. First, both synonymous mutations occur in a gene predicted to encode a permease subunit of an ABC transporter, and homologues of this transport system in P. aeruginosa and P. putida are glucose inducible and responsible for glucose uptake ( Fig. 2 ) [21] , [22] , [23] , [24] . Second, the benefits conferred are specific to glucose: neither mutation significantly affected fitness on alternate sugars ( Fig. 3 ). Third, from the same experiment, we identified a beneficial non-synonymous mutation (A10T) in gtsB that arose in an independently evolved population in glucose ( Figs 2a and 3 ), while populations selected in mannose or xylose never showed mutations in this gene. Finally, a gtsB knockout strain (Δ gtsB ) shows a significant fitness decrease in glucose of 14.23%±1.42 s.e.m. compared with the SBW25 ancestor ( t -test, df=7, P <0.0001; Fig. 3 ), but no significant difference in fitness from the ancestor on alternate sugars ( t -test, df=15, P =0.9563; Fig. 3 ). Taken together, these results strongly suggest that gtsB is a target of selection, that the synonymous mutations confer an adaptive advantage specifically on glucose and that the fitness gains do not stem from a loss of gene function. 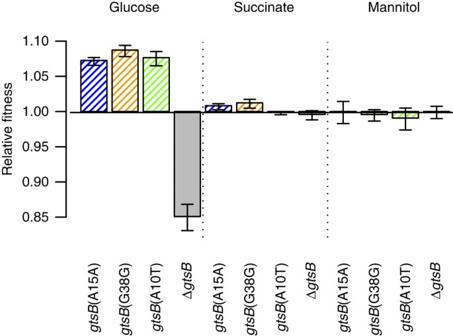Figure 3: Fitness effects ofgtsBmutations are specific to glucose. Fitness relative to the ancestor (SBW25) of genotypes containing the two synonymous mutations,gtsB(A15A) andgtsB(G38G), the non-synonymous mutation,gtsB(A10T), and thegtsBknockout, ΔgtsB, in glucose and two alternate carbon sources—succinate and mannitol. The mean±s.e.m. for each treatment is shown (n=8). Figure 3: Fitness effects of gtsB mutations are specific to glucose. Fitness relative to the ancestor (SBW25) of genotypes containing the two synonymous mutations, gtsB (A15A) and gtsB (G38G), the non-synonymous mutation, gtsB (A10T), and the gtsB knockout, Δ gtsB , in glucose and two alternate carbon sources—succinate and mannitol. The mean±s.e.m. for each treatment is shown ( n =8). Full size image Distribution of fitness effects In contrast to all previous work reporting fitness effects of synonymous mutations, the two we have uncovered arose spontaneously in an initially isogenic population and quickly went to near-fixation, a hallmark of strong positive selection. Indeed, our experimental results confirm that the fitness advantages of these mutations are large, and of similar magnitude to those reported for the first few non-synonymous mutations fixing in other microbial selection experiments (for example, see ref. 18 ). To provide further insight into the magnitude of the fitness effects associated with these mutations, we have examined the distribution of fitness effects fixed in other populations from the larger experiment [20] . Notably, the fitness effects of the synonymous mutations are well within the range of fitness effects for all other non-synonymous mutations evolving in these populations and are indistinguishable from the fitness effect of an independently isolated non-synonymous mutation in the same gene ( Fig. 4 ). The fitness effects of these synonymous mutations thus resemble those of any other non-synonymous mutation that has been selected. 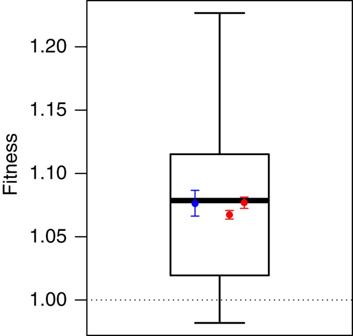Figure 4: Fitness effects of mutations fixing in SBW25 populations evolved under similar conditions20. Box and whiskers show the distribution of fitness effects of non-synonymous mutations. The box indicates the median, and the lower and upper quartiles (25 and 75%) of the data, while the whiskers indicate the minimum and maximum values (n=8). Red points show the fitness effects of the two synonymous mutations (A15A and G38G), and the blue point shows the fitness effect of a non-synonymous mutation (A10T) in the same gene (mean±s.e.m.,n=8). Figure 4: Fitness effects of mutations fixing in SBW25 populations evolved under similar conditions [20] . Box and whiskers show the distribution of fitness effects of non-synonymous mutations. The box indicates the median, and the lower and upper quartiles (25 and 75%) of the data, while the whiskers indicate the minimum and maximum values ( n =8). Red points show the fitness effects of the two synonymous mutations (A15A and G38G), and the blue point shows the fitness effect of a non-synonymous mutation (A10T) in the same gene (mean±s.e.m., n =8). Full size image Fitness advantage is caused by increased gene expression What is the mechanism by which the synonymous substitutions confer high fitness? As the amino-acid sequence is not changed, the mechanism presumably involves changes to gene expression at the level of transcription or translation, or perhaps even changes to protein secondary structure resulting from altered translation rates [4] , [6] , [7] . We obtained measures of gtsB gene expression by assaying transcript abundance using a luciferase reporter assay (see Methods and Supplementary Fig. 1 ). We found that the synonymous mutations and the independently evolved non-synonymous mutation in the same gene increased gene expression by approximately twofold in glucose ( Fig. 5a ; t -test, df=19, P <0.0001). Both the wild-type and mutant alleles were specifically expressed on glucose, indicating that there was no shift from inducible to constitutive expression. Although our assay cannot distinguish between an increase in gene expression due to increased rates of transcription or decreased rates of transcript degradation, we can confirm a link between increased gene expression and fitness. While transcriptional induction of the wild-type gtsB gene alone did not increase fitness, induction of the entire operon containing the gene was beneficial ( Fig. 5b and Supplementary Fig. 1 ). Taken together, these results indicate that increased expression of the ABC transporter operon is likely responsible for the increased fitness caused by these synonymous mutations. 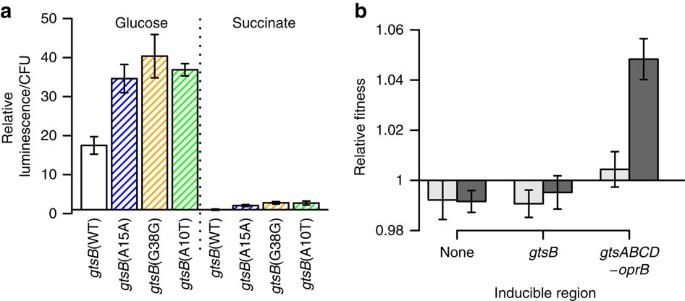Figure 5: The effects of thegtsBmutations on gene expression, and the effects of increased expression on fitness. (a) Reporter gene expression measured in luminescence/colony-forming units (CFU), relative to the minimum expression (mean±s.e.m.,n=5). Transcriptional reporter strains with the wild type (WT), synonymous (A15A and G38G) and non-synonymous (A10T) alleles ofgtsB-driving luciferase expression were tested in the selection environment (glucose) and with an alternate carbon source (succinate). (b) Mean fitness (±s.e.m.,n=11) of constructs containing inducible inserts. Light grey shows fitness in the absence of the inducer (IPTG) and dark grey shows fitness in the presence of the inducer. Figure 5: The effects of the gtsB mutations on gene expression, and the effects of increased expression on fitness. ( a ) Reporter gene expression measured in luminescence/colony-forming units (CFU), relative to the minimum expression (mean±s.e.m., n =5). Transcriptional reporter strains with the wild type (WT), synonymous (A15A and G38G) and non-synonymous (A10T) alleles of gtsB- driving luciferase expression were tested in the selection environment (glucose) and with an alternate carbon source (succinate). ( b ) Mean fitness (±s.e.m., n =11) of constructs containing inducible inserts. Light grey shows fitness in the absence of the inducer (IPTG) and dark grey shows fitness in the presence of the inducer. Full size image Synonymous mutations are often thought to impact both gene expression and fitness through modifications to codon usage bias, mRNA stability or protein folding, but these mechanisms seem unlikely explanations for our results. Both the A15A and the G38G mutations result in slightly less-preferred codons (see Methods and Supplementary Table 1 ), indicating that the increase in gene expression (and increase in fitness) cannot be due to aligning codon bias within the gene to that of highly expressed genes. Furthermore, previous studies suggest that codon bias must change by a substantial amount to have a measurable effect on gene expression [2] , much less fitness, and so the magnitude of the fitness effects seen here suggests a priori that codon bias is not a potential mechanism. Synonymous mutations can affect the stability of mRNA secondary structure through altered base pair interactions. Less stable secondary structures near a ribosomal binding site can lead to increases in mRNA and protein levels, presumably via more efficient translation initiation, while more stable structures can reduce expression levels [2] , [4] . Although the G38G mutation does decrease the predicted mRNA stability relative to the ancestor, the A15A mutation has no effect on predicted mRNA stability ( Supplementary Table 1 ), suggesting that changes in mRNA folding energy do not fully explain the effects of the substitutions. Changes to translational efficiencies caused by the synonymous mutations can result in altered protein folding [6] and could conceivably lead to increased fitness. This explanation seems unlikely given that increasing transcription of the wild-type allele increased fitness ( Fig. 5b ), however, further examination of this hypothesis must await a complete characterization of the GtsB protein. It is conceivable that the fitness benefit of these mutations comes via their interaction with regulatory factors that modulate transcription or translation. Two mechanisms seem plausible. First, the catabolite repression control (Crc) protein regulates glucose metabolism in Pseudomonads by binding to target mRNA and inhibiting translation [25] . If Crc binding to gtsB mRNA is inhibited by the synonymous mutations, this could result in increased GtsB expression. Although the gts operon is a predicted target of Crc [26] , deleting crc did not increase gene expression and fitness in the wild-type background and both remained elevated in the presence of the synonymous mutations ( Supplementary Fig. 2 ). Second, the synonymous mutations could prevent binding of a small RNA (sRNA) targeting the gtsB transcript for degradation [27] . However, we found that deleting hfq , a protein required for the activity of many sRNAs [28] , did not decrease the elevated levels of gene expression associated with the synonymous mutations ( Supplementary Fig. 3 ). That we find no empirical support for either of these models suggests that the molecular mechanism likely stems from effects of the synonymous mutations on binding an as-yet unidentified factor regulating transcript abundance through its effects on transcription rate or mRNA stability. Our results demonstrate unequivocally that synonymous mutations can increase fitness by amounts similar to that of non-synonymous mutations, and can play an important role in adaptive evolution. One potential criticism of our results is that they are not general or applicable to more natural, and presumably more complex, situations. Two observations argue against this view. First, as we noted above, we have confirmed that gtsB is a target of selection on glucose and that the synonymous mutations do not confer general fitness advantages to life in a laboratory environment. Any environment where selection favours the ability to grow on limiting glucose is thus likely to target mutations in gtsB , at least some of which could be synonymous. Second, comparative genomic evidence indicates that the synonymous mutations we have uncovered are the most common substitutions at those sites in closely related Pseudomonads ( Fig. 6 ). Taken together, these results suggest that these mutations may also be beneficial in more natural environments and are not just an artefact of life in a laboratory environment. 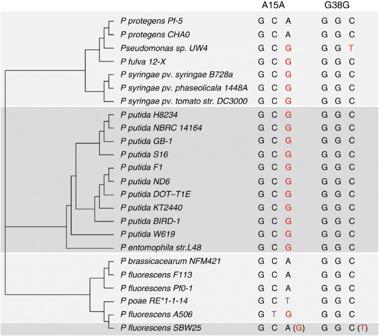Figure 6: Comparison of substitutions ingtsBat the locations of synonymous mutations A15A and G38G in 23 closely related species/strains ofPseudomonads. This comparison includes the BLAST (blastn) hits toP. fluorescensSBW25gtsBfor which the retrievedgtsBgene sequence did not differ in length from the querygtsBsequence. The phylogeny was constructed from full DNA sequences ofgtsB. Black letters indicate the same nucleotide as SBW25, red letters indicate the same nucleotide as an SBW25 synonymous mutant and grey letters indicate an alternate nucleotide. Figure 6: Comparison of substitutions in gtsB at the locations of synonymous mutations A15A and G38G in 23 closely related species/strains of Pseudomonads . This comparison includes the BLAST (blastn) hits to P. fluorescens SBW25 gtsB for which the retrieved gtsB gene sequence did not differ in length from the query gtsB sequence. The phylogeny was constructed from full DNA sequences of gtsB . Black letters indicate the same nucleotide as SBW25, red letters indicate the same nucleotide as an SBW25 synonymous mutant and grey letters indicate an alternate nucleotide. Full size image We have shown that the synonymous mutations identified in this study occur in a gene that is a target of selection, confer large fitness benefits typical of other non-synonymous mutations involved in adaptation to resource-limited environments, increase fitness via increased gene expression and are found in closely related species in nature. Moreover, it is notable that an independently isolated non-synonymous mutation in the same gene increases fitness by a comparable amount, displays the same resource specificity and shows a similar increase in gene expression as the synonymous mutations, suggesting that both types of mutations impact fitness by the same underlying mechanism. Synonymous mutations can thus contribute to adaptation and be positively selected. Synonymous mutations can therefore not always be assumed to be neutral in models that infer the strength of selection from comparative gene sequence data based on the relative rates of non-synonymous to synonymous mutations [4] . Rather, it seems more appropriate to treat the fitness effects of synonymous mutations in the same way as we do to other kinds of mutations, as draws from an underlying probability distribution of fitness effects that includes both deleterious and beneficial mutations. More generally, that we have uncovered an example of adaptive evolution driven by the substitution of two synonymous mutations in an experimental system evolving over a few hundred generations suggests that this class of mutation may be an underappreciated cause of adaptation and evolutionary dynamics in nature. Bacterial strains, plasmids and media The strains, plasmids and primers used in this study are listed in Supplementary Tables 2 and 3 . Plasmids were propagated in Escherichia coli DH5α or DH5αλpir (for pUIC3 derivatives). Transformation of DNA into E. coli and P. fluorescens was accomplished by chemical transformation, electroporation or conjugation according to standard protocols [29] , [30] . E. coli was grown on Luria broth (LB) media at 37 °C and P. fluorescens on LB or minimal (M9) media at 28 °C. The minimal media contained 48 mM Na 2 HPO 4 , 22 mM KH 2 PO 4 , 9 mM NaCl, 19 mM NH 4 Cl, 2 mM MgSO 4 and 0.1 mM CaCl 2 with either glucose (53 μM), succinate (80 μM) or mannitol (53 μM) as sole carbon source. Antibiotics were used at the following concentrations: 100 μg ml −1 ampicillin (Ap), 25 μg ml −1 kanamycin (Km) and 25 μg ml −1 gentamicin (Gm) for E. coli ; 100 μg ml −1 nitrofurantoin (Nf), 10 μg ml −1 tetracycline (Tc) and 10 μg ml −1 Gm for P. fluorescens . Media were supplemented with 5-bromo-4-chloro-3-indolyl-β-D-galactopyranoside (X-gal) at 20 μg ml −1 or isopropyl β-D-1-thiogalactopyranoside (IPTG) at 1 mM when appropriate. Selection experiment and competitive fitness assays As part of a larger experiment, we propagated an initially isogenic population of P. fluorescens SBW25- lacZ for 1,000 generations in a minimal medium containing glucose as a sole carbon source [20] . We estimated relative fitness of the population every 200 generations using 48 h head-to-head competitions against the SBW25 ancestor. Fitness was calculated as ω =( f final / f initial )^(1/doublings), where f initial and f final are the ratios of the frequency of the evolved population to the frequency of ancestral population before and after competition, respectively, and doublings refer to the number of doublings or generations that occur between the initial and final measurements. Fitness of the SBW25 allelic replacement constructs was estimated relative to SBW25- lacZ in glucose, succinate and mannitol environments to determine whether the detected fitness improvements were glucose specific. Whole-genome sequencing and genotyping Chromosomal DNA was extracted from the generation 1,000 population using a Promega Wizard Genomic DNA Purification kit and Illumina sequencing was performed by the Michael Smith Genome Sciences Centre. The sequence data were aligned to the P. fluorescens SBW25 reference genome NC_012660.1, and mutations were called and annotated using a custom computational pipeline [31] and BRESEQ [18] . The time dynamics of the detected mutations was characterized by isolating 24 colonies every 200 generations over the course of the experiment and amplifying a ~700-bp PCR product containing the putative single nucleotide polymorphism (SNP) from each isolate. PCR products were directly sequenced by the McGill University and Genome Quebec Innovation Centre. We probed for the large 35,107 bp deletion in each isolate by characterizing them as motile (ancestral state) versus non-motile (evolved state) on semi-solid agar plates, a trait associated with this deletion. Allelic replacement constructs The gtsB synonymous mutations (A15A and G38G) were individually introduced into SBW25 using a previously described allelic exchange method involving the pUIC3 vector [32] , [33] . PCR fragments containing the mutations and 1-kb of flanking sequence on each side were amplified using primers 4845-BglII-F and 4845-AvrII-R from chromosomal DNA isolated from the evolved bacteria. The DNA was digested with BglII and AvrII and cloned into the compatible BglII and SpeI sites of pUIC3 to generate pUIC3-A15A and pUIC3-G38G. The plasmids were mobilized into SBW25 by triparental mating with the help of pRK2013. Exconjugates carrying the plasmid integrated by a single homologous recombination were selected on LB agar with Nf and Tc. To allow for plasmid excision by a second homologous recombination, bacteria were grown for two 24 h subcultures in LB broth, and plated on LB agar containing X-gal [32] . The rare white colonies do not express pUIC3-encoded lacZ and were screened for tetracycline sensitivity to verify loss of the plasmid backbone. The gtsB locus of independent white colonies was sequenced to identify clones with the desired SNPs. Additional gtsB mutations (A10T and Δ gtsB ) and the crc (PFLU5989) and hfq (PFLU0520) deletions were recombined into P. fluorescens using a pUIC3 derivative in which the lacZY genes were replaced by the sacB counterselectable marker. This vector was generated by excising the lacZY genes from pUIC3 by EcoRI digestion, followed by self-ligation, transformation into DH5αλpir and screening for white colonies on LB with Ap and X-gal. A 2-kb fragment containing the sacB gene was amplified from pEX18Tc [34] using primers SacB-EcoRI and SacB-MfeI and inserted at the EcoRI site of the lacZY -excised pUIC3. The resulting plasmid (pAH79) confers sucrose sensitivity, Ap r and Tc r . Transcription of the sacB gene is oriented towards the multiple cloning site, which carries an additional unique EcoRI site suitable for cloning. The pAH79 derivative containing the gtsB (A10T) mutation was generated by amplifying the 2-kb gtsB locus using primers 22F-5324097 and 22R-5324097 from DNA isolated from an evolved clone carrying the mutation. The fragment was digested with BglII and XbaI and cloned into the BglII and SpeI sites of pAH79 to generate pAH79-A10T. The gtsB deletion plasmid was constructed by amplifying 1-kb fragments upstream and downstream of the gtsB gene with primer pairs 4845-del-F1/R1 and 4845-del-F2/R2. The two products were digested and ligated together using engineered SacI sites, and the 2-kb hybrid product was amplified with primers 4845-del-F1/R2. The resulting fragment contains a gtsB allele with an in-frame deletion of codons 7 through 274 (of 302 total codons). The fragment was digested with BamHI and XbaI and inserted in the compatible BglII and SpeI sites of pAH79 to generate pAH79-Δ gtsB . The crc and hfq deletion plasmids (pAH79-Δ crc and pAH79-Δ hfq ) were generated similarly with primer pairs specific to crc (crc-del-F1/R1 and crc-del-F3/R3) and hfq (hfq-del-F1/R1 and hfq-del-F2/R2). The crc allele contains a deletion of codons 31 to 216 (of 259 total), with a stop codon introduced after codon 31. The hfq allele carries a deletion of codons 8 to 82 (of 86 total). Chromosomal integration of the pAH79 derivatives in P. fluorescens was achieved by triparental mating as described for the pUIC3 constructs. sacB counterselection enabled selection for the second recombination event by streaking Tc r exconjugates on LB agar containing 5% sucrose. Sucrose-resistant colonies were tested for T c sensitivity and screened for the presence of the desired mutations by sequencing (SNPs) or a PCR test (deletions). Transcriptional luciferase fusions Gene expression of the gtsB alleles was examined using transcriptional luciferase fusions delivered by a site-specific mini-Tn7 transposon [35] . A 2.1-kb PCR fragment including the 350-bp gtsA promoter region, gtsA open reading frame and 115 codons (out of 302) of the gtsB open reading frame was amplified with primers 4845-lacZ-F1 and 4845-lacZ-R1. The fragment was digested with XmaI and XhoI and ligated at the corresponding sites of the vector pUC18-mini-Tn7T-Gm- lux . The truncated gtsB′ open reading frame encounters a vector-encoded stop codon 36 nucleotides downstream of the XhoI site, and the start codon of the initial lux gene is located 432 nucleotides further. Reporter constructs containing four gtsB alleles (wild type, A15A, G38G and A10T) were introduced into P. fluorescens by co-electroporation with the pTNS2 helper plasmid by a previously described method [36] , with selection on LB Gm 10 (for SBW25) or LB Gm 1 (for SBW25 Δ crc ). The Δ hfq reporter constructs were generated by deleting the hfq gene from the SBW25 reporter constructs. Insertion at the att Tn7 locus was verified as recommended [35] by PCR amplification with mini-Tn7- and SBW25-specific primer sets (PTn7R/PglmS-up-SBW25 and PTn7L/PglmS-down-SBW25). Activity of the transcriptional fusions was determined in exponential phase liquid cultures. Overnight cultures grown in M9-glucose or M9-succinate media were diluted (1:100) in 1.5 ml fresh media and incubated 7 h with shaking in 24-well plates. Luminescence at 520 nm was measured using a microplate reader (Tecan Infinite 200 Pro). The luminescence values were standardized by cell density, determined by dilution plating. Inducible gene expression constructs Regulated expression of gtsB and gtsABCD-oprB by the P tac promoter was achieved using mini-Tn7T-LAC constructs [35] . A 1-kb fragment containing the gtsB open reading frame and 53-bp of upstream sequence was amplified with primers SacI-F2-Tac and XhoI-R1-Tac, digested with SacI and XhoI and cloned into the corresponding sites of pUC18-mini-Tn7T-LAC to generate pAH308. The 5.8-kb gtsABCD-oprB fragment was amplified with primers SacI-F1-Tac and NheI-R3-Tac and included sequences from 31-bp upstream of the gtsA start codon to 32-bp downstream of the oprB stop codon. The product was digested with SacI and NheI and cloned into the compatible SacI and SpeI sites of pUC18-mini-Tn7T-LAC to generate pAH305. Transposition of the expression constructs to the SBW25 att Tn7 site was performed as described for the luciferase fusions. The fitness effects of inducing the gtsB and gtsABCD-oprB genes were measured via 48 h head-to-head competitions against SBW25- lacZ mini-Tn7T-LAC under inducing (1 mM IPTG) and non-inducing (no IPTG) conditions. Codon bias estimates and mRNA structure comparisons To look for potentially important changes in codon bias as a result of the two synonymous mutations, we compared the codon usage of highly expressed genes in SBW25 to codon usage within the gtsB gene using the codon adaptation index [37] . We used the SBW25 ribosomal protein genes as our sample of highly expressed genes. To calculate change in codon adaptation index caused by each mutation, we used the ‘cai’ function in the ‘seqinr’ package [38] in R. We used ‘mfold’ [39] to predict and compare mRNA structure and stability of the ancestral gtsB gene and the three mutated versions. Accession codes: The gtsB gene (PFLU4845) sequences reported in this paper have been deposited in the GenBank nucleotide database under the accession codes KJ787789 to KJ787791 . How to cite this article: Bailey, S. F. et al. Adaptive synonymous mutations in an experimentally evolved Pseudomonas fluorescens population. Nat. Commun. 5:4076 doi: 10.1038/ncomms5076 (2014).